Electron uptake by iron-oxidizing phototrophic bacteria Oxidation–reduction reactions underlie energy generation in nearly all life forms. Although most organisms use soluble oxidants and reductants, some microbes can access solid-phase materials as electron-acceptors or -donors via extracellular electron transfer. Many studies have focused on the reduction of solid-phase oxidants. Far less is known about electron uptake via microbial extracellular electron transfer, and almost nothing is known about the associated mechanisms. Here we show that the iron-oxidizing photoautotroph Rhodopseudomonas palustris TIE-1 accepts electrons from a poised electrode, with carbon dioxide as the sole carbon source/electron acceptor. Both electron uptake and ruBisCo form I expression are stimulated by light. Electron uptake also occurs in the dark, uncoupled from photosynthesis. Notably, the pioABC operon, which encodes a protein system essential for photoautotrophic growth by ferrous iron oxidation, influences electron uptake. These data reveal a previously unknown metabolic versatility of photoferrotrophs to use extracellular electron transfer for electron uptake. Microbial metabolic activity substantially influences matter and energy flow through the biosphere and drives global biogeochemical cycles [1] . Microorganisms have broad metabolic capabilities and can use chemically diverse, soluble substrates for energy generation. Some microbes can also use solid-phase electron acceptors and -donors via a process called extracellular electron transfer (EET) [2] , [3] , [4] , [5] . Recent years have been a watershed for microbial EET, with many studies focusing on the relevance of EET in bioremediation and biotechnology [6] , [7] . Although studies over the past few decades have examined the role of microbial EET in donating electrons to metal oxides and oxygen [6] , [8] , [9] , [10] , the involvement of microbial EET in facilitating electron uptake has come to the fore only recently [11] . Studies show that mixed microbial communities facilitate cathodic reactions in bioelectrochemical systems (BESs), implicating microbes in electron uptake [11] . Recent studies using pure cultures have shown that at least three microbes are capable of taking up current from an electrode: Sporomusa ovata [12] , Mariprofundus ferrooxydans PV-1 (ref. 13 ) and Shewanella oneidensis MR-1 (ref. 14 ). Only the study performed on Shewanella considered the genetic loci to be likely involved in electron uptake [14] . As such, the mechanisms underlying electron uptake by microbes including Shewanella remain poorly understood. Characterizing how microbes take up electrons from solid-phase electron donors is critical to our understanding of the ecological and evolutionary implications of this process, as well as to any future biotechnology efforts such as electrosynthesis [6] , [15] . The establishment of genetic, genomic and metabolic studies in microbes that naturally take up electrons via EET will lead to the following: (1) identification of the associated genetic determinants; (2) the underlying molecular mechanisms; and (3) also facilitate experiments that examine the relationship between electron uptake and cellular metabolism. Here we present data on our studies of Rhodopseudomonas palustris TIE-1 (TIE-1), a photoautotrophic microbe capable of accepting electrons from a variety of electron donors, including iron [16] , [17] , [18] ( Supplementary Fig. 1 ). We chose TIE-1 as the model organism because it uses ferrous iron, Fe(II), as an electron donor for photosynthesis (photoferrotrophy) [16] . Moreover, the metabolic versatility and genetic tractability of TIE-1 helps to readily interrogate the fundamental physiological relevance of electron uptake, including the degree and conditions under which TIE-1 takes up electrons, some genetic loci encoding systems involved in electron uptake, and the relationship between electron uptake and other physiological processes such as photosynthesis and carbon fixation. We observe that TIE-1 accepts electrons from a poised electrode, with carbon dioxide as the sole carbon source/electron acceptor. Both electron uptake and ruBisCo (ribulose-1, 5-bisphosphate carboxylase/oxygenase) form I expression are stimulated by light. Electron uptake also occurs in the dark, uncoupled from photosynthesis. The pioABC operon, which encodes a protein system essential for photoautotrophic growth by ferrous iron oxidation, influences electron uptake. TIE-1 accepts electrons from a poised electrode To characterize electron uptake by TIE-1, BESs were used. BESs are experimental systems where an electrode is submerged in a bioreactor and is used to mimic the midpoint potential of solid-phase minerals [3] , [6] . BESs provide an attractive alternative to using natural redox active minerals, allowing one to study microbial EET without confounding issues such as mineralogical changes during experimentation [6] , [9] , [13] , [19] , [20] . The electrodes were poised at +100 mV versus Standard Hydrogen Electrode (SHE) ( Supplementary Fig. 2 ), as this potential is consistent with forms of Fe(II) used by TIE-1 (ref. 21 ). TIE-1 was subjected to three treatments as follows: (1) illuminated reactors with poised electrodes passing current (illuminated treatment); (2) non-illuminated reactors with poised electrodes passing current (dark treatment); and (3) illuminated reactors with electrodes at open circuit, passing no current (control treatment). The highest rates of current uptake by the TIE-1 wild-type (WT) were observed in illuminated treatments, up to ~1.5 μA cm −2 ( Fig. 1a ). Cyclic voltammetry (CV) of the electrodes in the illuminated treatments revealed two modest but discernable cathodic peaks at +0.27 and +0.4 V (versus SHE) in the WT, which were absent in the abiotic control ( Fig. 1b ), suggesting the presence of redox active components in the illuminated reactors. Cathodic current was also observed in the dark treatments, suggesting that current uptake occurred under these conditions, although ~70% lower than when illuminated ( Fig. 1a ). We observed that cells were attached to electrodes during all biotic treatments, with the highest viable cell densities occurring in the light treatment ( Fig. 2a,b , Supplementary Fig. 3 , Supplementary Tables 1 and 2 ). Planktonic cell numbers increased during the course of the 1-day incubations, although the increase in the WT illuminated and control treatments were not significantly different at the end of these experiments ( Supplementary Tables 3 and 4 ). 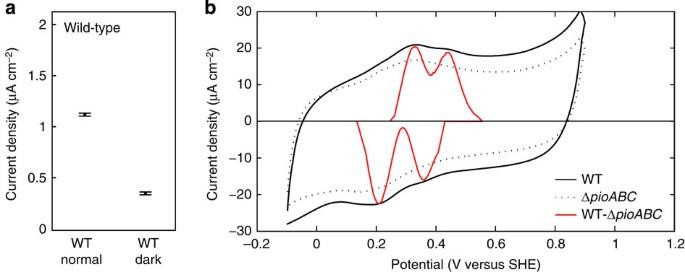Figure 1: Current uptake by WTR. palustrisTIE-1. (a) Current densities ofR. palustrisTIE-1 WT under illuminated and dark conditions. Error bars indicate s.d. of these averages (n=3), and data reported are consistent with 10 independent runs. (b) Cyclic voltammograms of WT and ΔpioABCmutant after 96 h of treatment in bioelectrochemical reactors with electrodes poised at +100 mV versus SHE. Two sets of anodic–cathodic peak pairs were identified at 0.27 and 0.40 V, respectively. The red trace depicts the difference in magnitude between the WT and the ΔpioABCmutant strain. Figure 1: Current uptake by WT R. palustris TIE-1. ( a ) Current densities of R. palustris TIE-1 WT under illuminated and dark conditions. Error bars indicate s.d. of these averages ( n =3), and data reported are consistent with 10 independent runs. ( b ) Cyclic voltammograms of WT and Δ pioABC mutant after 96 h of treatment in bioelectrochemical reactors with electrodes poised at +100 mV versus SHE. Two sets of anodic–cathodic peak pairs were identified at 0.27 and 0.40 V, respectively. The red trace depicts the difference in magnitude between the WT and the Δ pioABC mutant strain. 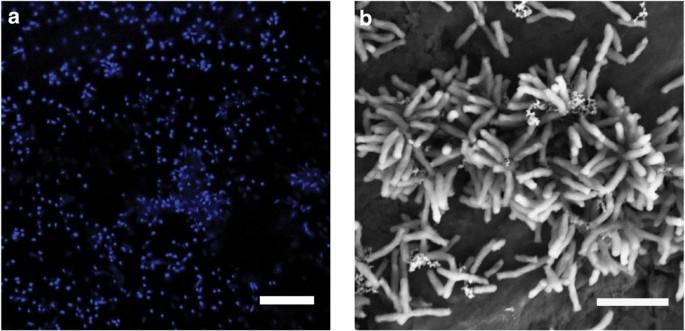Figure 2:R. palustrisTIE-1 cells attached to cathodes. (a) Fluorescence micrographs of aR. palustrisTIE-1 WT-illuminated biofilm. Scale bar, 10 μm. (b) Scanning electron micrograph of a WT-illuminated biofilm. Scale bar, 3 μm. Full size image Figure 2: R. palustris TIE-1 cells attached to cathodes. ( a ) Fluorescence micrographs of a R. palustris TIE-1 WT-illuminated biofilm. Scale bar, 10 μm. ( b ) Scanning electron micrograph of a WT-illuminated biofilm. Scale bar, 3 μm. Full size image To best capture the changes in gene expression during the onset of EET, these treatments lasted ~24 h to avoid issues that can arise during prolonged experiments (for example, differences in growth phase). Nevertheless, the apparent changes in planktonic cell density would suggest that (1) current was being used to support planktonic growth; or (2) an exogenous electron donor was available for growth. Notably, in separate 5-day illuminated treatments, TIE-1 exhibited 10-fold higher densities than dark and control treatments. However, in these shorter-term illuminated treatments, mass balance calculations suggest that the planktonic cell increase in the bioreactors is two orders of magnitude lower than that predicted if all current went to biomass ( Supplementary Note 1 ). Moreover, the trace concentrations of iron present in the medium (to support biosynthesis) could only account for up to 4.0 × 10 4 cells per ml of the observed cell increase (for calculations see Supplementary Note 2 ). Thus, there is an electron sink other than biomass, and notably the gene expression data suggest that this could be reductive CO 2 assimilation (discussed in detail below). These data provide the first evidence of light-stimulated electron uptake by a photoferrotroph, with some electron uptake also occurring in the dark, independent of photosynthesis. Phototrophic microbes related to TIE-1 use photic energy for ATP synthesis through cyclic electron flow, without the need for an electron donor [22] . An electron donor is only required to produce reducing equivalents (NADPH) for cellular metabolism most likely by reverse electron transfer [23] . In the dark, no ATP can be generated via photosynthesis but cellular metabolism continues [22] , thus requiring an electron donor that is likely represented by the observed dark current in our experiments. The dark current also suggests that the electron uptake machinery is independent (or can be uncoupled) of the cyclic photosynthetic apparatus. The increase in electron uptake in the presence of light suggests that the ATP generated using the energy of light is used by cellular processes, necessitating a higher level of electron uptake. The pioABC operon has a role in electron uptake Because these data reveal that TIE-1 accepts electrons from a solid-phase conductor, we reasoned that it might use conserved strategies to mediate this electron uptake. Previous studies have shown that pioABC is essential for photoferrotrophy, and have speculated that the Pio proteins might be involved in electron transfer from Fe(II) to the electron transport chain [17] , [21] . The pioABC operon encodes the putative proteins PioA, a periplasmic decaheme cytochrome, PioB, an outer membrane porin, and PioC, a periplasmic high potential iron–sulfur cluster protein [17] , [21] ( Supplementary Fig. 4 ). Using mutant studies and expression analysis, we directly tested whether the PioABC system has a role in electron uptake. We observed that Δ pioABC -illuminated biofilms accepted 30% less current than the WT ( Fig. 3a ), and the mutant illuminated biofilms were ~8–10-fold less dense than the WT ( Supplementary Table 2 ). Fewer ΔpioABC mutants colonized the electrode in the illuminated treatments, which might result from an attachment defect. However, this was not observed in the control treatments, that is, in the absence of current, as the mutant cell densities were comparable to the WT ( ΔpioABC: 9.2 × 10 6 cells per cm 2 ; WT: 8.1 × 10 6 cells per cm 2 ). 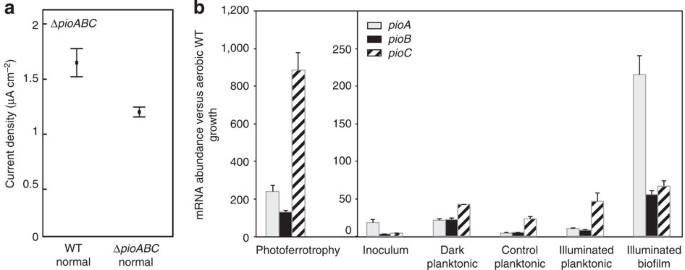Figure 3: Current uptake and mRNA abundance of thepioABCoperon by WTR. palustrisTIE-1 andΔpioABCmutant under various conditions. (a) Current densities ofR. palustrisTIE-1 WT andΔpioABCmutant under illuminated conditions. Error bars indicate s.d. of these averages (n=3), and data are consistent with 10 independent runs. (b)pioABCgene transcript abundance determined in the WT grown photoautotrophically on hydrogen and 5 mM FeCl2. qRT–PCR data are the averages ±s.e. for three biological replicates assayed in triplicate. Figure 3: Current uptake and mRNA abundance of the pioABC operon by WT R. palustris TIE-1 and ΔpioABC mutant under various conditions. ( a ) Current densities of R. palustris TIE-1 WT and ΔpioABC mutant under illuminated conditions. Error bars indicate s.d. of these averages ( n =3), and data are consistent with 10 independent runs. ( b ) pioABC gene transcript abundance determined in the WT grown photoautotrophically on hydrogen and 5 mM FeCl 2 . qRT–PCR data are the averages ±s.e. for three biological replicates assayed in triplicate. Full size image If we assume that only attached cells contribute to electron uptake, then the Δ pioABC mutants seem to accept more current per cell than the WT ( Supplementary Tables 5 and 6 ). This would imply that the Δ pioABC mutant cells can take up electrons more actively, perhaps via compensatory changes. We posit, however, that such an assumption is inaccurate. as it disregards the potential contribution of planktonic cells to electron uptake ( Supplementary Fig. 2 ). Regardless, these data collectively show that the Pio system influences electron uptake, although other mechanisms of electron uptake clearly exist in TIE-1, as the mutant maintains nearly 70% of the current uptake seen in the WT ( Fig. 3a ). Future studies should examine the means by which the Pio system influences both phototrophic iron oxidation and EET, and its potential role in governing attachment to poised electrodes. We hypothesized that electron uptake might influence physiological systems that have a role in EET as well as redox balance. Accordingly, we assessed the expression of the target genes, including those encoding the PioABC proteins, across all treatments. Expression of pioA in the WT-illuminated biofilm was upregulated by ~48-fold, whereas pioB and pioC showed more modest upregulation compared with the control treatment (11- and 3-fold, respectively; Fig. 3b ). The observed levels of pioA in the WT-illuminated biofilm were well above those of the inoculum (grown on H 2 :CO 2 ; Fig. 3b ). They were, however, comparable to gene expression observed during photoferrotrophic growth on soluble Fe(II) in conventional culture apparatus. The decreased current uptake of the Δ pioABC mutant as well as the observed upregulation of the Pio genes in the BES system together suggest that the PioABC proteins may be involved in electron uptake by TIE-1 under these conditions. It should be noted that the PioABC module occurs in a number of anoxygenic phototrophic microbes, which might show light-enhanced electron uptake as observed in TIE-1 ( Supplementary Table 7 ), Moreover, non-phototrophic ferrous iron-oxidizing bacteria (FeOB) also possess the PioAB module, raising the question as to whether these organisms perform light-independent electron uptake similar to the observed dark current in TIE-1. The involvement of the MtrAB (related to PioAB [17] ) system in the electron acceptance by S. oneidensis (MR-1) from a poised electrode also suggests that this module might have a direct role in electron uptake [14] . Electron uptake stimulates expression of other genes We used expression analyses and microscopy to further examine TIE-1’s response to electron uptake. Exopolysaccharide ( eps ) genes were highly upregulated in the WT-illuminated biofilms and, in some cases, in the Δ pioABC -illuminated biofilms. Expression analysis further showed that the pioC homologue (another high potential iron–sulfur cluster protein located elsewhere on the chromosome) was upregulated (fourfold) in the WT-illuminated planktonic cells (cells not attached to the electrode present in the medium) compared with the control treatment ( Fig. 4A(b) ), suggesting that the encoded protein might have a role in planktonic cell increase under these conditions. Microscopy revealed that EPS production was most abundant in illuminated biofilms ( Fig. 4A(a) and B(a) ; Supplementary Fig. 5a,b ). Protein staining established the presence of extracellular proteins in the cells attached to the electrodes ( Supplementary Fig. 5c,d ). Future analysis on biofilm and planktonic cells and the produced EPS will help determine the role of these elements in electron uptake. 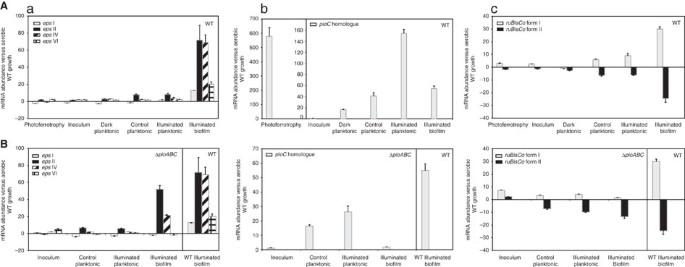Figure 4: mRNA abundance determined in theR. palustrisTIE-1 WT (A) and ΔpioABC(B). (a) Exopolysaccharide (eps) genes; (b)pioChomologue; and (c)ruBisCoform I and II mRNA abundance. Cell were grown photoautotrophically on hydrogen and 5 mM FeCl2. qRT–PCR data are the averages ±s.e. for three biological replicates assayed in triplicate.eps I=Rpal_3203,eps II=Rpal_3763,eps IV=Rpal_3771,eps VI=Rpal_3777,pioChomologue=Rpal_4085. Figure 4: mRNA abundance determined in the R. palustris TIE-1 WT ( A ) and Δ pioABC ( B ). ( a ) Exopolysaccharide ( eps ) genes; ( b ) pioC homologue; and ( c ) ruBisCo form I and II mRNA abundance. Cell were grown photoautotrophically on hydrogen and 5 mM FeCl 2 . qRT–PCR data are the averages ±s.e. for three biological replicates assayed in triplicate. eps I =Rpal_3203, eps II =Rpal_3763, eps IV =Rpal_3771, eps VI =Rpal_3777, pioC homologue=Rpal_4085. Full size image ruBisCo form I expression increases during electron uptake Previous studies have shown that in organisms related to TIE-1, electron donors are required for generation of reducing equivalents, namely NAD(P)H, which serves as a reductant for cellular processes such as carbon fixation via the Calvin cycle [22] , [24] , [25] , [26] . RuBisCo, a key enzyme in the Calvin cycle, assimilates CO 2 into ribulose-1,5-bisphosphate yielding two molecules of 3-phosphoglycerate, which are eventually reduced by NAD(P)H to glyceraldehyde 3-phosphate in the reductive phase of the cycle [24] , [25] , [26] . TIE-1 and related microbes harbour genes encoding two forms of ruBisCo : forms I and II (refs 24 , 25 , 26 ). We observed that ruBisCO form I was most highly expressed in WT-illuminated biofilms ( Fig. 4A(c) ), and was typically higher than ruBisCo form II during conventional, photoautotrophic growth on hydrogen and Fe(II) ( Fig. 4A(c) ). Notably, ruBisCo form I expression was not induced in the dark treatment ( Fig. 4A(c) ). Previous studies on the regulation of ruBisCo form I expression in CGA009/10 (~99% identity to TIE-1 (ref. 16 )) show that it is under exquisite control and is positively regulated by ATP and NAD(P)H, metabolites that indicate the energy status of the cell [27] . During electron uptake in the presence of light, TIE-1 likely produces abundant ATP and NAD(P)H, which we posit leads to the increase in ruBisCo form I expression. In contrast, both these metabolites are likely lower in the dark, and thus ruBisCo form I expression decreases. It has also been suggested that RuBisCo form I can indirectly act as an electron sink (because increase in its expression leads to higher production of 3-phosphoglycerate, which serves as the substrate for the reductive part of the Calvin cycle) to maintain redox balance in photosynthetic bacteria related to TIE-1 (refs 25 , 26 ). Our data provide a first glimpse on the ability of the photoautotrophic bacterium R. palustris TIE-1 to accept electrons from a solid-phase electron donor. Because photoautotrophs are exposed to diurnal cycles of light and dark conditions, we tested the effect of illumination on the ability of TIE-1 to accept electrons. Our results show that TIE-1 accepts electrons under both light and dark conditions, although light strongly stimulates electron acceptance ( Fig. 1a ). The massive upregulation in genes that encode for the pioABC system (encoding proteins that are suggested to have a critical role in phototrophic iron oxidation by TIE-1 (ref. 17 )), as well as the decrease in current observed in pioABC mutants, imply that the Pio proteins are engaged in electron uptake. In contrast, the pioABC mutants appear to have an attachment defect to poised electrodes, thus exhibiting higher cell-specific electron uptake rates compared with the WT ( Fig. 3a , Supplementary Tables 2 and 6 ). This apparent pleiotropy makes it difficult to ascribe a simple role to the pioABC system in electron uptake. It should be noted that our experimental design does not allow us to exclude the possibility that both the biofilm and the planktonic cells were engaged in electron uptake, and the free living and biofilm lifestyles might be dynamic ( Supplementary Fig. 2 ). The planktonic cells may have contributed to current uptake through direct encounters with the electrode (these reactors were well stirred) or via soluble compounds (we were unable, however, to detect any redox active compounds in the spent medium; Supplementary Figs 2 and 6 ). Transcriptomic analysis showed that ruBisCo form I expression was highest in the poised illuminated electrodes ( Fig. 4A(c) ), suggesting that this enzyme could be an indirect electron sink as has been observed in other related organisms [25] , [26] . Because RuBisCo is part of the Calvin Cycle, the carbon fixation pathway in TIE-1, it is plausible that some of these electrons would go to biomass. Although we did see an increase in the total cell density, there was no significant difference among these short-term treatments, and the mass balance analyses suggest that biomass only accounts for a modest amount of the total current passed ( Supplementary Tables 1–4 ). As mentioned, these experiments were designed to be short in duration to avoid confounding factors associated with growth and changes in growth phase. In light of TIE-1’s typically modest growth rates, it is likely that increases in biomass attributable to electron uptake during these short-term treatments are below our limits of resolution. In nature, electron uptake via EET could ameliorate metabolic dilemmas that neutrophilic FeOBs, such as TIE-1, are known to face. FeOBs often contend with the precipitation of insoluble iron oxides outside the cell that are a byproduct of their metabolic activity and potentially limit Fe(II) availability [21] , [28] . TIE-1 produces poorly crystalline Fe(III) hydroxides, which over time are abiotically transformed to the (semi)conductive minerals goethite and magnetite [16] , [29] . Conduction of electrons through this matrix would allow TIE-1 (and potentially other FeOBs) access to electrons from remote electron donors, including Fe(II) ( Supplementary Fig. 7 ), via processes such as electron conduction and iron atom exchange [30] , [31] , [32] . Indeed, recent studies have shown that conductive minerals can facilitate electron transfer to microbes from remote electron donors (including other microbes) [33] . These data extend this phenomenon to photoautotrophs that is highly relevant because their restriction to the photic zone might hinder access to reductants in deeper, anaerobic layers [22] , [34] . In addition to the ecological advantages of electron uptake via EET, there is substantial interest in exploiting photoautotrophs for both energy and biofuel generation [11] , and identifying a genetically tractable photoautotroph that can use electric current as an electron donor holds promise in future electrosynthesis applications [11] . Although the ecological significance of EET is just coming to the fore, our data illustrate the potential value of EET to microorganisms in nature, in particular photoautotrophs. Bacterial strains, media and growth conditions R. palustris TIE-1 was grown as described previously [18] . For experiments, cells were pre-grown autotrophically on 80% hydrogen:20% carbon dioxide (H 2 :CO 2 ) at 200 kPa in freshwater medium (FW) with 20 mM bicarbonate. The Δ pioABC strain used herein was constructed as previously described [17] . Phototrophic pre-growth was at 30 ° C using a 60-W incandescent light source providing total irradiance of ~40 W m −2 . Bioelectrochemical reactor studies were conducted with FW medium (minimal salts medium lacking any added electron donors [16] , [17] , [18] ) with 20 mM bicarbonate (sole carbon source [16] , [17] , [18] ), buffered to pH 6.8 and with no exogenous electron donor. All bacterial strains were routinely tested for purity by standard PCR using primers indicated in Supplementary Table 8 . Owing to biological variation in the cultivation effort, which resulted in different cell densities in the inoculum and prohibits comparison across treatments, we ran a WT control in parallel with every individual treatment to account for these differences. All comparisons between WT and treatments are made using these paired runs. BES and conditions The BESs consisted of new, acid-washed, combusted 350 ml borosilicate glass H-cell reactors equipped with two butyl rubber sampling ports in the cathodic chamber (Adams and Chittenden Scientific Glass, Berkeley, CA, USA). A vacuum clamp held the anodic and cathodic chambers together, and electrolytes were separated using a cation-exchange membrane (Nafion 117) with an active cross-section of 20 cm 2 (Fuel Cell Store, Boulder, CO, USA). The working electrodes consisted of spectroscopically pure 1/8′′-diameter graphite evaporation rods (SPI 01685-FA, Structure Probe Inc., West Chester, PA, USA) that were mechanically polished with 1200 grit sandpaper, soaked in 5% HCl for 12 h and stored in ultrapure deionized water. The graphite rods were thoroughly dried before use by allowing the water to evaporate. Each reactor was fitted with three graphite rods to provide a total immersed projected electrode surface area of 18 cm 2 . The rods were sealed with fittings and ferrules on the reactor cap (Upchurch Scientific, Oak Harbor, WA, USA). Outside the reactor, rods were electrically connected to one potentiostat using alligator clips (described below). The counter electrode consisted of carbon cloth (Fuel Cell Store), which was mechanically attached to a titanium wire pierced through a rubber stopper (VWR) and suspended in the counter chamber. Electrical conditions and cyclic voltammograms The reactors were poised using custom-built potentiostats engineered for microbial chronoamperometry (Karma Electronics Inc., Somerville, MA, USA). Data were collected through a National Instruments DAQ (NI-6225) every 10 s using Labview SignalExpress software (National Instruments, Austin, TX, USA). Based on preliminary analyses of electroactivity in WT R. palustris TIE-1, the reactors were poised at +100 mV versus SHE (−100 mV of the biological E pc roughly at +200 mV versus SHE) to assure cathodic conditions during the experiment. Importantly, this potential also ensures that a reductive Fe(III)/Fe(II) cycle is not established during these experiments (the redox potential at pH 7.0 of the Fe(III)/Fe(II) couple is +14 mV, and electron transfer from an electrode poised at +100 mV will be an endergonic process) [15] . Reported current densities (μA cm −2 ) were obtained by averaging regions of >8 h of stable current in each reactor. CV was conducted using a Gamry R600 potentiostat (Gamry, Warminster, PA, USA). Biofilm CVs were obtained with a scan range of −100 to +900 mV versus SHE at a rate of 20 mV per second. Supernatant voltammograms were obtained using a 3-mm diameter glassy carbon electrode (part no. A-002012, BioLogic, Claix, France), under a N 2 atmosphere, scanned between 0 and +500 mV versus SHE at 20 mV per second. We were unable to detect any electro-active soluble species in the 0.2-mM filtered spent medium ( Supplementary Fig. 7 ). To assess the active surface area variability between electrodes, CVs were collected abiotically in FW medium. Potential is referenced to the SHE unless otherwise specified. Description of bioelectrochemical setups The distance between the working and counter electrodes was ~11 cm. Assembled BES reactors were sterilized by autoclaving in sterilization pouches and placed inside an anaerobic chamber (Coy, 2% hydrogen and palladium catalysts). Ag/AgCl reference electrodes were custom-made using glass tubing (4 mm KIMAX), silver wire (0.5 mm diameter) and porous vycor tips (1/8′ diameter, MF-2064, BASi). Reference electrodes were calibrated before each experiment, placed in the anaerobic chamber, sterilized with 70% ethanol and placed in the counter chamber for the duration of the experiments. Although inside the anaerobic chamber, media and counter buffer were added to the cathode and anode chambers, respectively. Inoculation of the BESs occurred inside the anaerobic chamber before transferring them outside the anaerobic chamber to establish electrical connections. The reactor system was purged continuously with a 1-cm 3 min −1 stream of 0.2 μm filter-sterilized, deoxygenated gas stream of 80%:20% N 2 :CO 2 and 100% N 2 on the cathodic and anodic side, respectively, using a hypodermic needle immersed 1 cm below the media surface. The gases were deoxygenated using a high capacity oxygen trap lowering the oxygen levels to <0.01 p.p.m. (Restek, Bellefonte, PA, USA). Each BES was individually housed with a fresh incandescent 60 W bulb providing a total irradiance of ~40 W m −2 . Dark BESs lacked a bulb and were covered thoroughly with black paper to prevent light exposure. All working chambers were stirred gently with a magnetic bar and incubated at 30 ° C. All incubations, across all treatments, lasted 24 h. Sampling The reactors were inoculated with 10 ml of cells in the mid-exponential phase of photoautotrophic growth on 80% H 2 : 20% CO 2 . Media (1 ml) was withdrawn from the reactors immediately following inoculation and used for optical density (OD 660 ) determination with a 4802 spectrophotometer (Cole Parmer, Vernon Hills, IL, USA), and for pH measurements (Inlab Expert Pro pH metre and probe; Mettler Toledo, Schwerzback, Switzerland). Culture (4 ml) was also withdrawn from the reactors for cell counts. Cells were fixed in 4% paraformaldehyde for cell counting (Electron Microscopy Sciences, Hatfield, PA, USA). At the end of each experiment, one of the electrodes was immediately dipped into RNA later (Qiagen, Valencia, CA, USA) for RNA extraction. Also, 5 ml of planktonic cells were immediately preserved in RNA later and filtered on a polyethersulfone membrane for RNA extraction (Corning, Tewksbury, MA, USA). All RNA samples were stored at −80 ° C. A second electrode was cut into ~5 mm pieces and transferred into fixatives or staining solutions for microscopic analyses (described below). Post experimentation, 1 ml of planktonic cells was sampled for OD 660 determination, and 2–4 ml for pH measurements. The remaining culture volume was then filtered on a 0.2-μm cellulose acetate filter (Corning). After resuspension in 8 ml of media, these planktonic cells were pelleted in two 2 ml microcentrifuge tubes (18,000 g for 10 min) and kept at −80 °C along with the filtered spent medium. Protein analysis Subsamples for total protein analysis were processed in Prot loBind 1.5 or 2 ml microcentrifuge tubes (Eppendorf, Hauppauge, NY, USA). Trichloroacetic acid precipitation was used as previously described [18] . The pellets were dried under vacuum for 1 h to remove residual acetone and then resuspended in 650 μl of 3 M Urea (ACS grade, Alfa-Aesar, Ward Hill, MA, USA). To ensure complete resuspension, the samples were incubated at 80 °C for 3 days with frequent sonication in a sonic bath (FS30H; Thermo Fisher Scientific, Waltham, MA, USA). The Pierce BCA (bichinchoninic acid) Protein Assay Kit (Thermo Scientific, Rockford, IL, USA) was used using the microtiter plate method for protein estimation as specified by the manufacturer with the provided bovine serum albumin as the standard protein. Each sample was quantified in triplicate. Absorbance at 562 nm was measured after 30 s shaking at 37 °C using a Spectramax Plus 384 plate reader (Molecular Devices, Sunnyvale, CA, USA). Fluorescence microscopy sample preparation and imaging Sections of the electrode were placed into one of three solutions containing 1 μM 4′,6-diamidino-2-phenylindole (Life Technologies, Grand Island, NY, USA) as well as (1) LIVE/DEAD stain (0.5 μM SYTO 9 and 3 μM propidium iodide, L7012, Life Technologies); (2) EPS stain (200 mg l −1 Concanavalin A and Alexa 488, Life Technologies); and (3) Protein stain (undiluted FilmTracer SYPRO Ruby Biofilm Matrix Stain, Life Technologies). Tubes were wrapped in aluminium foil and kept at room temperature for at least 30 min. Samples were then placed in 1 × phosphate-buffered saline (PBS) in a glass-bottomed dish and imaged with a Zeiss 700 inverted confocal microscope with the following imaging lasers and Zeiss filters: (1) live/dead=555 and 488 nm, SP490; 405 nm, SP555; (2) EPS=488 and 405 nm, SP490 and LP490; and (3) protein=555 nm, SP 490; 405 nm, SP555. This work was performed at the Harvard Center for Biological Imaging. Scanning electron microscopy Sections of the electrode were cut using sterile techniques and immediately placed into a sterile microcentrifuge tube containing one of three solutions: (1) 5% glutaraldehyde (Electron Microscopy Sciences) in 1 × PBS; (2) 2% paraformaldehyde (Electron Microscopy Sciences) in 1 × PBS; and (3) 2% glutaraldehyde in 1 × PBS with 0.15% Safranin O (Sigma-Aldrich, St Louis, MO, USA), which has previously been shown to aid in EPS preservation [7] . Samples were held at 4 °C for 24 h before being subjected to ethanol dehydration by placing them in 35, 50, 70, 95 and 100% ethanol (200 proof) in PBS or 0.1 M PBS solutions for 10 min each. The 100% ethanol solution was changed five times, and the sample was left in ethanol for critical point drying (Autosamdri 815A; Tousimis, Inc.) with a 15-min purge time. The samples were adhered to scanning electron microscopy (SEM) posts with carbon film tape and then imaged with a SEM at 5 kV (JEOL, Inc.). Cell counts for electrode samples were performed by analysing microscopy fields taken at the same working distance (4.5 mm) to image, counting at least 500 cells or examining 12 fields of view if cell density was low and normalized to total area. This work was performed at the Harvard Center for Nanoscale Systems (CNS). RNA isolation For planktonic assessments, preserved cells were dislodged from the polyethersulfone membrane before RNA extraction by vortexing for 3 min in a Tris-EDTA buffer. For biofilm assessment, the cells were dislodged from the graphite by scraping with a sterile razor, then vortexing vigorously in Tris-EDTA buffer. RNA was extracted as described previously [5] . The RNA concentration was quantified using a NanoDrop ND1000 (Thermo Scientific, Wilmington, DE, USA). RNA amplification The RNA obtained from the biofilm on the graphite was cleaned with the MEGAclear Kit (Life Technologies) as per the manufacturer’s guidelines. The purified RNA was precipitated using ammonium acetate. The reconstituted RNA was used as template for the MessageAmp II-Bacteria Kit as per the manufacturer’s guidelines (Life Technologies). Quantitative reverse transcription PCR Gene expression analysis was performed using quantitative reverse transcription PCR (qRT–PCR). The comparative Ct method was used as described previously to assess expression of the pioABC operon and other relevant genes [5] . Primer efficiencies were determined using the manufacturer’s method (Applied Biosystems, Inc. User Bulletin no. 2). clpX and recA were used as the two internal standards, which have been previously used and validated as internal standards [18] . The primers used for the assays are indicated in Supplementary Table 5 . The iScript cDNA synthesis kit was used for reverse transcription (Bio-Rad, Hercules, CA, USA). The iTaq FAST SYBR Green Supermix with ROX (Bio-Rad) and the Stratagene Mx3005P QPCR System (Agilent, Santa Clara, CA, USA) were used for all quantitative assays. Cell counting The paraformaldehyde-fixed samples were transferred into Amicon centrifuge filters (Amicon Ultrael 100k, regenerated cellulose membrane; Millipore, Carrigtwohill, CO, Ireland) and centrifuged for 10 min at 1,000 g . The pellet was resuspended in PBS and washed twice. The cells were recovered by centrifugation of the Amicon in reverse position for 15 min at 3,000 g . The resulting samples had <0.04% paraformaldehyde. Picogreen was added to the cells (Quant-iT PicoGreen dsDNA, Life Technologies), and the cells were counted in 96-well plates along with 50 μl of Sphero AccuCount blank beads (Spheroteck, Lake Forest, IL, USA). Cell density was estimated with a LSRII flow cytometer (BD, Sparks, MD, USA) using a 488-nm laser. A calibration curve relating the ratio of cell events to beads events with cell density was constructed by analysing a dilution series of a cell sample, the density of which has been determined by microscopy (with a Helber Bacteria Cell counting chamber with Thoma ruling, Hawksley, Lancing, Sussex, UK). Inductively coupled plasma mass spectrometry To measure the concentration of iron present in FW medium inductively coupled plasma mass spectrometry (ICP-MS) was performed using an Agilent 7700x ICP-MS with an octopole MS (Agilent). Internal standards used were Germanium and Manganese, which were within the detection limit of our system. The amount of iron in the basal medium was 4 μM and ranged from 2–4 μM in the spent medium. In silico methods For identifying homologues of the PioABC proteins, delta-blast [35] , FASTA [36] ( http://www.ebi.ac.uk/Tools/sss/fasta/ ), and the IMG ortholog neighbourhood search was used [37] ( http://img.jgi.doe.gov/cgi-bin/w/main.cgi ). Sequence similarity was calculated using EMBOSS matcher [38] , [39] ( http://www.ebi.ac.uk/Tools/psa/emboss_matcher/ ). The data reported is accurate as of October 2nd, 2012. How to cite this article: Bose, A. et al. Electron uptake by iron-oxidizing phototrophic bacteria. Nat. Commun. 5:3391 doi: 10.1038/ncomms4391 (2014).